Sulfenate anions as organocatalysts for benzylic chloromethyl coupling polymerization via C=C bond formation Organocatalytic polymerization reactions have a number of advantages over their metal-catalyzed counterparts, including environmental friendliness, ease of catalyst synthesis and storage, and alternative reaction pathways. Here we introduce an organocatalytic polymerization method called benzylic chloromethyl-coupling polymerization (BCCP). BCCP is catalyzed by organocatalysts not previously employed in polymerization processes (sulfenate anions), which are generated from bench-stable sulfoxide precatalysts. The sulfenate anion promotes an umpolung polycondensation via step-growth propagation cycles involving sulfoxide intermediates. BCCP represents an example of an organocatalyst that links monomers by C=C double bond formation and offers transition metal-free access to a wide variety of polymers that cannot be synthesized by traditional precursor routes. Innovations in polymer chemistry and materials science often have their genesis in the introduction of small molecule catalysts [1] , [2] . This is particularly true in the developing field of organocatalytic polymerization chemistry. [3] , [4] Organocatalytic polymerization reactions have a number of advantages over their metal-catalyzed counterparts, including environmental friendliness, reduced toxicity and cost, ease of catalyst synthesis and storage, and access to alternative reaction pathways. Furthermore, organocatalysts circumvent problems caused by metal residue contamination of polymers, which can severely limit biomedical and electronic applications, and complicate polymer purification and processing [3] , [4] . The majority of organocatalytic polymerizations involve ring-opening polymerizations using cyclic esters, carbonates, ethers, siloxanes, anhydrides, and phosphoesters [4] . Herein we introduce a class of organocatalytic polymerization processes termed benzylic chloromethyl-coupling polymerization (BCCP). BCCP represents the application of sulfenate anion organocatalysts to polymerization processes. The sulfenate anion-catalyzed process proceeds via an umpolung mechanism and represents a rare example of an organocatalysts that enchains monomers by C=C bond formation [5] , [6] . Design of BCCP is validated in the context of poly( m -phenylene vinylene) (P m PV) synthesis. In this study, P m PV’s with M n as high as 17,400 Da and with very high trans -selectivity are obtained. To demonstrate the mechanistic distinctness of BCCP, a non-conjugated polymer bearing quaternary –C(CF 3 ) 2 spacers between stilbene units in the polymer backbone is synthesized. Moreover, two alternating co-polymers as representatives of poly[(1,3-phenylene vinylene)-alt-arene]s and poly[(1,3-phenylene vinylene)-alt-(1,4-phenylene vinylene)] (P m PV p PV)s are synthesized. Nuclear magnetic resonance (NMR) spectra, thermal, photophysical, electrochemical, and charge transport properties of the above mentioned co-polymers are characterized. The polymers reported herein cannot be prepared by classic precursor routes (Gilch, Wesling, and Vanderzande methods). Design of the BCCP Sulfenate anions (ArSO – ) are highly reactive intermediates in biological chemistry and in organic reactions [7] , [8] , [9] , [10] . We recently disclosed that sulfenate anions can act as organocatalysts and reported their ability to catalytically dehydrocouple benzyl halides under basic conditions to yield trans -stilbenes (Fig. 1a ) [11] and their application to catalytic cross-coupling of benzyl chlorides with benzaldehyde derivatives to produce diarylacetylenes [12] . The efficiency of sulfenate anion catalysts in these reactions, and their high selectivity for formation of trans -stilbenes, inspired us to explore their potential in polymerization reactions. We hypothesized that substrates bearing two benzylic chloromethyl groups would be suitable monomers for polymerization. The benzylic chloromethyl substituents could be located on the same aromatic system or on different aromatic rings separated by linking groups, as represented in Fig. 1b . Fig. 1 Sulfenate anion-catalyzed reactions. a Dehydrocoupling of benzyl chlorides to produce stilbenes. b Generic representation of the benzylic chloromethyl-coupling polymerization (BCCP), where the blue box represents an aromatic system or tethered aromatic rings. c Fundamental steps in the organocatalytic BCCP Full size image Based on this hypothesis, we designed the 1,3-bis(chloromethyl)benzene monomer A (Fig. 1c ). We envisioned that the sulfenate anion would react with monomer A via an S N 2 reaction to generate sulfoxide B . In the presence of base, sulfoxide B is reversibly deprotonated to generate carbanion C . Anion C is a reactive nucleophile and undergoes S N 2 with monomer A to form the first C–C bond. Base promoted E2 elimination of intermediate D provides dimer E and liberates the sulfenate anion to further catalyze the polycondensation of E . Notably, the product is a P m PV, which is an important class of organic semiconductors with applications in optoelectronics, such as organic light-emitting diodes (OLEDs), solar cells, organic lasers, sensors, and displays [13] , [14] , [15] , [16] , [17] , [18] . Although the synthesis of PPV’s has been developed, including precursor routes [19] , [20] , [21] , [22] , [23] , olefin metathesis polymerizations [23] , nucleophilic condensations [24] , [25] , [26] , [27] , [28] , [29] , and cross-coupling polymerizations [30] , [31] , [32] , [33] , [34] , [35] , [36] , to the best of our knowledge this is a unique organocatalytic method for the synthesis of this important class of polymers. Moreover, P m PV is a challenging target, because meta -linkages preclude formation of quinodimethane intermediates, prohibiting classic PPV precursor routes (Gilch, Wesling and Vanderzande methods) [33] , [37] , [38] , [39] , [40] . Optimization of BCCP with monomer M1 Starting from the optimized coupling of benzyl chlorides used in our stilbene synthesis (Fig. 1a ) [11] , we selected cyclopentyl methyl ether (CPME) as solvent and KO t Bu as base at 80 o C, to optimize the polymerization of monomer M1 (Fig. 2 ). A long alkyl chain was introduced onto the P m PV backbone to assure the resulting polymer P1 has good solubility in common organic solvents. Initial reactions were conducted in 24-well plates on 10 µmol scale by adapting small molecule high-throughput experimentation (HTE) [41] , [42] , [43] , [44] , [45] , [46] , [47] , [48] techniques to polymerizations (see Supplementary Method, High-Throughput Experimentation screenings for polymerization for full details). As shown in Fig. 2a , we initially focused on air-stable benzylic sulfoxide catalysts ( 1 – 9 ) ArSOCH 2 Ph with various Ar–S groups and one precatalyst ( 10 ) with 4 catalyst loadings (10, 7.5, 5.0, and 2.5 mol %). Reactions were heated for 24 h at 80 o C followed by cooling and work up by addition of 10 µL of water and removal of the volatile materials. Next, CHCl 3 was added to each well to dissolve the products followed by cold methanol to precipitate the solid polymer. Finally, filtration of the solid, dissolution in tetrahydrofuran (THF) and analysis by gel permeation chromatography (GPC) against polystyrene standards were performed. In this screen we observed complete polymerization at 10, 7.5, and 5.0 mol % catalyst loadings. There was little impact of the substituents on the aryl ring of the sulfenate anion (ArSO – ), with similar M n and polydispersity index (PDI) ( M n ~ 10,000 were observed at 10 and 7.5 mol % loading and M n ~ 9000 at 5.0 mol % loading). 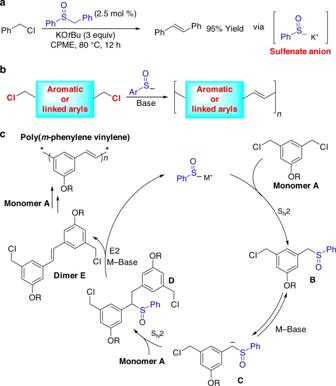Fig. 1 Sulfenate anion-catalyzed reactions.aDehydrocoupling of benzyl chlorides to produce stilbenes.bGeneric representation of the benzylic chloromethyl-coupling polymerization (BCCP), where the blue box represents an aromatic system or tethered aromatic rings.cFundamental steps in the organocatalytic BCCP Lower catalyst loadings of 2.5 mol % led to oligomerization (see Supplementary Table 1 ). Moreover, we observed complete consumption of monomer M1 after 10 min. A rapid loss of monomer at the beginning of the polymerization indicates that the BCCP proceeds by a step-growth mechanism. Fig. 2 Optimization by HTE Screening. a Precatalysts employed leading to sulfoxide 10 for further studies. b Additional base screen indicated that NaN(SiMe 3 ) 2 ( M n = 10,200) gave the best results, but lower than KO t Bu ( M n = 10,900) of panel a . c Additional solvent screen, wherein MTBE gave the best results ( M n = 13,200) higher than CPME of panel a . See Supplementary Table 3 for all results Full size image At this stage of our investigations we chose to employ precatalyst 10 . 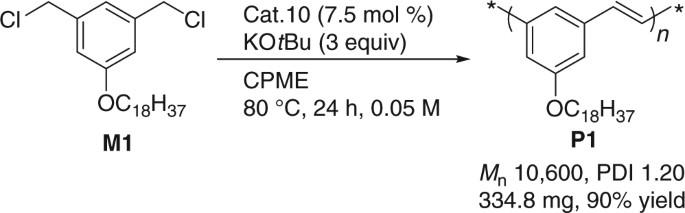Fig. 3 Scale-up ofP1. Synthesis ofP1by BCCP reaction Under the basic conditions of the polymerization, 10 rapidly undergoes E2 elimination to form styrene and generate the sulfenate anion [12] . The most promising results with precatalyst 10 were with 7.5 mol % ( M n 10,900, PDI 1.26). At this loading, we conducted a second screen focused on 10 bases [LiO t Bu, NaO t Bu, LiN(SiMe 3 ) 2 , NaN(SiMe 3 ) 2, KN(SiMe 3 ) 2 , NaH, KH, KOSiMe 3 , KOPh, NaOMe] under otherwise identical conditions (Fig. 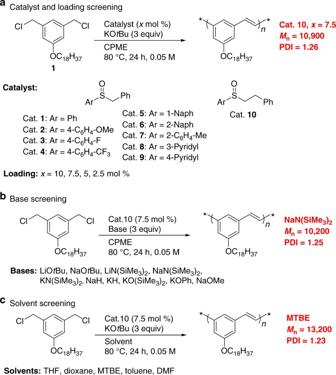2b ). Fig. 2 Optimization by HTE Screening.aPrecatalysts employed leading to sulfoxide10for further studies.bAdditional base screen indicated that NaN(SiMe3)2(Mn= 10,200) gave the best results, but lower than KOtBu (Mn= 10,900) of panela.cAdditional solvent screen, wherein MTBE gave the best results (Mn= 13,200) higher than CPME of panela. See Supplementary Table3for all results Analysis of the resulting reactions indicated that polymer was obtained only with LiN(SiMe 3 ) 2 , NaN(SiMe 3 ) 2, KN(SiMe 3 ) 2 with M n all lower than with KO t Bu from the first screen (see Supplementary Table 2 ). The next step in the optimization was a solvent screen. We examined five solvents (THF, dioxane, MTBE (methyl tert -butyl ether), toluene, and dimethylformamide). As shown in Fig. 2C , the most promising result was obtained in MTBE ( M n 13,200, PDI 1.23). After narrowing our optimization parameters to precatalyst 10 (7.5 mol %), KO t Bu, and CPME and MTBE as two top solvents, we conducted lab-scale (0.1 mmol) polymerizations to validate the microscale results and further optimize the BCCP (Table 1 ). Lab-scale polycondensation of monomer M1 with both CPME and MTBE at 0.05 M concentration yielded polymer with M n 10,400, PDI 1.28 in 91% isolated yield for CPME and polymer with M n 13,600, PDI 1.21 in 69% isolated yield with MTBE. The results confirmed that M n and PDI of polymers obtained at 10 µmol scale could be reproduced at 0.1 mmol scale. With CPME as solvent, increasing concentration to 0.1 M and 0.2 M (entries 3–4) led to higher M n (11,200 at 0.1 M and 12,200 at 0.2 M) with similar PDIs. The yields, however, dropped from 91% (0.05 M) to 86% (0.1 M) and 73% (0.2 M). With MTBE as solvent, increasing concentration led to higher M n of 15,300 (0.1 M, entry 5) in 72% yield and 17,400 (0.2 M, entry 6) in 71% yield, with PDI of the corresponding polymers of 1.41. Employing 4 and 5 equivalents of KO t Bu afforded polymer product with similar M n , PDI, and yield (entries 7–8). The M n dropped to 10,200 when 6 equiv. of base were employed (entry 9). Table 1 BCCP optimization Full size table Scalability of BCCP with monomer M1 Scalability is an important attribute of polymerization catalysts. We next scaled the BCCP of M1 to 1 mmol scale using the conditions outlined in Table 1 , entry 1. Under the reaction conditions shown in Fig. 3 , the polymer P1 was obtained with M n 10,600 and PDI 1.20 in 90% yield (334.8 mg). Fig. 3 Scale-up of P1 . Synthesis of P1 by BCCP reaction Full size image Mechanistic distinctness of BCCP Traditionally, PPVs were synthesized by a two-step quinodimethane polymerization/elimination protocol (the precursor route) [19] . The quinodimethane polymerization forms a non-conjugated polymer that is then converted to the conjugated PPV by high-temperature (180–300 o C) thermal elimination reaction (Fig. 4a ) [49] . The harsh conditions required for converting non-conjugated precursor polymers to PPVs and the incomplete elimination lead to structural defects, which affect the luminescence quantum efficiency of the PPV films [50] . In sharp contrast, sulfenate anion-catalyzed BCCP proceeds by a different mechanism, which results in chemoselective construction of trans double bonds (Fig. 4b ). Compared with other common methods for the preparation of PPVs such as transition metal-mediated Heck reactions, cross-coupling reactions, and metathesis reactions [51] , BCCP is a transition metal-free process. Fig. 4 Comparison of BCCP polymerization with precursor routes. a Summary of precursor route. b BCCP polymerization Full size image To highlight the advantage of BCCP over precursor routes (Gilch, Wesling, and Vanderzande methods) (Fig. 4a ), we designed monomer M2 in which two benzyl chloromethyl groups are linked by a C(CF 3 ) 2 bridge (Fig. 5 ). As the C(CF 3 ) 2 linker prevents the formation of quinodimethane intermediate, polymer P2 could not be prepared by precursor routes (Fig. 4a ). Using the conditions in Table 1 (entry 1), the BCCP afforded polymer P2 in 82% yield with M n 14,300 and PDI 1.45. Fig. 5 Synthesis of polymer P2 . The polymer generated has a C(CF 3 ) 2 linker Full size image Synthesis and characterization of alternating 1,3- and 1,4-linked copolymers It is well-known that OLED device performance is greatly influenced by the structural regularity of the polymers. To further demonstrate the synthetic potential of BCCP, we next employed BCCP in the synthesis of challenging alternating copolymers. We designed a class of monomers ( M3 , Fig. 6a ) by incorporating a flourenyl group between two meta -phenyl groups. Polymerization of monomer M3 bearing different central Ar groups is expected to lead to a new class of structurally regular and alternating poly[(1,3-phenylene vinylene)-alt-arene]s. As proof-of-concept, we synthesized a fluorine-containing monomer M3-1 . BCCP of M3-1 led to co-polymer P3-1 in 91% yield with M n 13,000 and PDI 2.00 (see Supplementary Method, 1 mmol Scale synthesis and characterization of co-polymer P3-1 , P4-1 , for the synthesis of monomer M3-1 and co-polymer P4-1 ). Fig. 6 Design and synthesis of alternating co-polymers. a Poly[(1,3-phenylene vinylene)-alt-arene]s. b Poly[(1,3-phenylene vinylene)-alt-(1,4-phenylene vinylene)] (P m PV p PV)s Full size image Previous studies have shown that (P m PV p PV)s are highly photoluminescent polymers with well-defined conjugation lengths [52] , [53] , [54] , [55] . Such observations inspired us to design a member of this class, monomer M4 . We expect that polymerization of M4 type monomers will achieve the synthesis of structurally regular (P m PV p PV)s with 1:1 alternating m PV and p PV units along the chain linked by trans C=C bonds (Fig. 6b ). Moreover, incorporation of different moieties as side-chains into the P m PV p PV backbone (R group on the p PV unit of P4 ), would allow tuning of the emission wavelength, emission color and change the quantum efficiency of the resulting co-polymer P4 . As a proof-of-concept, we synthesized a thiophene-containing monomer M4-1 . BCCP of M4-1 led to co-polymer P4-1 in 93% yield with M n 8000 and PDI 1.82 (see Supplementary Method, 1 mmol Scale synthesis and characterization of co-polymer P3-1 , P4-1 , for the synthesis of monomer M4-1 and co-polymer P4-1 ). Notably, both polymers P3-1 and P4-1 are not accessible by the precursor route, demonstrating the value of BCCP in co-polymer synthesis. The thermal, photophysical, electrochemical and charge transport properties of P3-1 and P4-1 were characterized (see Supplementary Figure 37 ). As shown in Fig. 7a , I, the decomposition temperatures ( T d , corresponding to 5% weight loss) measured from thermogravimetric analysis were 420 o C and 404 o C for P3-1 and P4-1 , respectively, indicating good thermal stability. Thermal stability is valuable for long device operation in emission materials [15] . From the glass transition temperatures ( T g ) observed from differential scanning calorimetry (DSC) for the more rigid fluorene containing P3-1 was 141 o C; however, no obvious phase transition temperature could be obtained for P4-1 with more flexible C–C double bonds in the conjugated backbone (Fig. 7b ). Both polymers showed bright emission under UV excitation, as shown in the photo images of Fig. 7c,d , II. From the UV-Vis spectra in both solution and film (Fig. 7c,d ), it is found that two-dimensional conjugated P4-1 with the pendant thiophene ring exhibited broader and red-shifted absorption relative to P3-1 , with a one-dimensional conjugated polymer backbone. Regarding the photoluminescence (PL), the thiophene-containing P4-1 displayed red-shifted PL compared with P3-1 , with emission peaks in the deep blue (435 nm in THF and 457 nm in the film state) for P4-1 and ultra-violet (373 nm in THF and 402 nm in the film state) for P3-1 . The electrochemical properties were measured by cyclic voltammetry (Fig. 7e ). Both polymers exhibited quasi-reversible oxidation and irreversible reduction behavior. The highest occupied molecular orbital (HOMO) and lowest unoccupied molecular orbital (LUMO) energy levels were determined from the onset of oxidation and reduction curves for P3-1 and P4-1 , and were calculated to be −5.97/−2.60 eV and −5.65/−2.77 eV, respectively. Compared with P3-1 , the introduction of a strong electron-donating thiophene ring in P4-1 significantly raises the HOMO level by 0.32 eV, suggesting a more efficient hole-injection and better hole transport properties of P4-1 in optoelectronic devices. This prediction is in good agreement with the measured hole mobility from the space charge limited current method (Fig. 7f ). The hole mobility for the thiophene-containing P4-1 is estimated to be 1.56 × 10 −6 cm 2 V −1 s −1 , which doubles P3-1 of 7.79 × 10 −7 cm 2 V −1 s −1 . Fig. 7 Polymer characterization. a TGA curves of the co-polymers P3-1 and P4-1 . b DSC curves of the co-polymers P3-1 and P4-1 . c Normalized UV-Vis absorption and PL spectra of co-polymers P3-1 and P4-1 in THF solution and photographs of polymer photoluminescence under 365 nm light in THF solution. d Normalized UV-Vis absorption and PL spectra of co-polymers P3-1 and P4-1 in film state and photographs of polymer photoluminescence under 365 nm light in solid state. e Cyclic voltammograms of the oxidation curves in dichloromethane and reduction curves in THF for co-polymers P3-1 and P4-1 . f Current density–voltage ( J – V ) characteristics of hole-only devices with structure of ITO/PEDOT:PSS(30 nm)/ P3-1 or P4-1 (30 nm)/MoO 3 (8 nm)/Ag Full size image 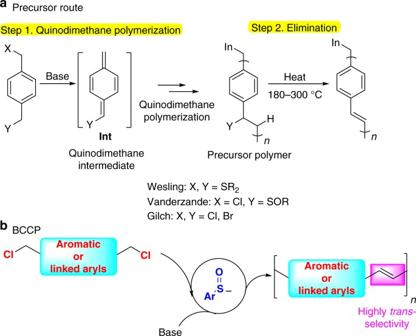Fig. 4 Comparison of BCCP polymerization with precursor routes.aSummary of precursor route.bBCCP polymerization Introduced herein is a class of organocatalytic polymerization processes termed BCCP. The organocatalysts for this process, sulfenate anions, are operationally trivial to generate from bench-stable sulfoxide precatalysts in the presence of base. Sulfenate anion organocatalysts are unique in that they enable generation of C=C double bonds of the type found in PPV’s and other stilbene-based polymers. We demonstrated the application of sulfenate anion-catalyzed transfer polycondensation methods to polymers bearing isolated stilbene motifs. The important conceptual advance of this work is that it suggests that small organic molecules that can activate substrates via nucleophilic attack, acidify neighboring hydrogens leading to umpolung reactivity, and then behave as leaving groups can be considered in polymerization processes to forge C=C linkages. From the synthetic aspect, BCCP offers transition metal-free access to wide varieties of polymers that cannot be synthesized by traditional precursor routes (Gilch, Wesling, and Vanderzande methods). To further demonstrate the synthetic potential of BCCP, two alternating co-polymers were synthesized as representatives of classes of poly[(1,3-phenylene vinylene)-alt-arene]s and (P m PV p PV)s. NMR spectra, thermal, photophysical, electrochemical, and charge transport properties of the above mentioned polymers were characterized. Further studies are underway to apply BCCP to the preparation of novel functionalized polymers. General procedure for the 0.1 mmol BCCP An oven-dried 8 mL microwave vial equipped with a stir bar was charged with monomer M1 (44.4 mg, 0.10 mmol) under a nitrogen atmosphere in a glove box. A solution of precatalyst 10 (1.73 mg, 0.0075 mmol) in 1.0 mL anhydrous CPME was added by syringe. Next, a solution of KO t Bu (33.6 mg, 0.30 mmol) in 1.0 mL anhydrous CPME was added by syringe. The reaction was stirred for 24 h at 80 °C, quenched with 2 drops of H 2 O via syringe, cooled to room temperature, and opened to air. After the volatile materials were removed with a rotary evaporator, CHCl 3 (2 mL) was added into each vial and the slurry solution was allowed to stir for 10 min. Cold methanol (6 mL) and H 2 O (0.5 mL) was then added into each vial to precipitate the polymer and the slurry solution with polymer suspension was allowed to stir for 10 min. The mixture was then transferred with a pipette onto a Whatman autovial syringeless filter (5 mL, 0.45 µm polytetrafluoroethylene (PTFE) membrane). After the MeOH/CHCl 3 /H 2 O solution was filtered, polymer that remained in the filter was washed sequentially with 5 mL MeOH and 5 mL pentane. Finally, the polymer remaining in the filter was transferred into a 20 mL vial with spatula and dried under vacuum to yield a pale yellow solid in 33.8 mg, 91% yield. 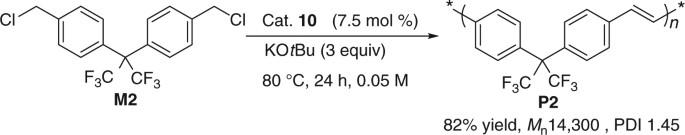Fig. 5 Synthesis of polymerP2. The polymer generated has a C(CF3)2linker General procedure for the scale-up (1 mmol) polymerization An oven-dried 100 mL Schlenk tube equipped with a stir bar was charged with monomer 1 (444.0 mg, 1.0 mmol) and precatalyst 10 (17.3 mg, 0.075 mmol). The Schlenk tube was sealed with a rubber septum and was connected to a Schlenk line, evacuated, and refilled with nitrogen (repeated three times). Next, a solution of KO t Bu (336 mg, 3.0 mmol) in 20 mL anhydrous CPME was added by syringe. The reaction was stirred for 24 h at 80 °C, cooled to room temperature, opened to air, and quenched with 1 mL of H 2 O. The reaction mixture was firstly transferred to a 250 mL round-bottom flask and the volatile materials were removed with a rotary evaporator. Next, CHCl 3 (20 mL) was added into flask and the slurry solution was allowed to stir for 10 min. Cold methanol (60 mL) was added into the flask to precipitate the polymer and the slurry solution with polymer suspension was allowed to stir for 10 min. The mixture was then filtered on a glass fritted filter funnel (75 mL). After the MeOH/CHCl 3 solution was filtered, the resulting solid was washed with H 2 O (5 mL), MeOH (20 mL *3), and pentane (5 mL). 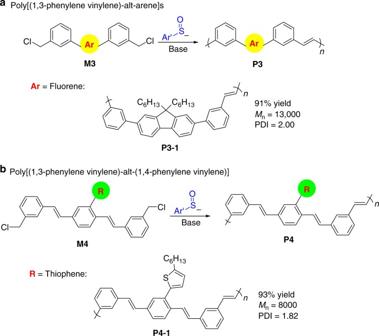Fig. 6 Design and synthesis of alternating co-polymers.aPoly[(1,3-phenylene vinylene)-alt-arene]s.bPoly[(1,3-phenylene vinylene)-alt-(1,4-phenylene vinylene)] (PmPVpPV)s 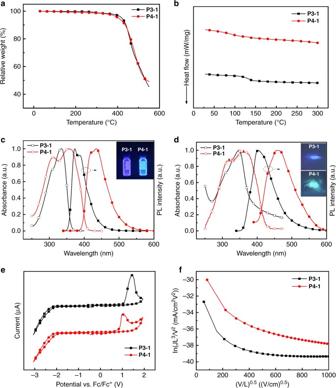Fig. 7 Polymer characterization.aTGA curves of the co-polymersP3-1andP4-1.bDSC curves of the co-polymersP3-1andP4-1.cNormalized UV-Vis absorption and PL spectra of co-polymersP3-1andP4-1in THF solution and photographs of polymer photoluminescence under 365 nm light in THF solution.dNormalized UV-Vis absorption and PL spectra of co-polymersP3-1andP4-1in film state and photographs of polymer photoluminescence under 365 nm light in solid state.eCyclic voltammograms of the oxidation curves in dichloromethane and reduction curves in THF for co-polymersP3-1andP4-1.fCurrent density–voltage (J–V) characteristics of hole-only devices with structure of ITO/PEDOT:PSS(30 nm)/P3-1orP4-1(30 nm)/MoO3(8 nm)/Ag The solid was collected and dried in a vacuum as pale yellow solid to provide 334.8 mg, 90% yield of the polymer. Data availability The authors declare that the data supporting the findings of this study are available within the article and its Supplementary Information files.